Bose–Einstein condensation in an ultra-hot gas of pumped magnons Bose–Einstein condensation of quasi-particles such as excitons, polaritons, magnons and photons is a fascinating quantum mechanical phenomenon. Unlike the Bose–Einstein condensation of real particles (like atoms), these processes do not require low temperatures, since the high densities of low-energy quasi-particles needed for the condensate to form can be produced via external pumping. Here we demonstrate that such a pumping can create remarkably high effective temperatures in a narrow spectral region of the lowest energy states in a magnon gas, resulting in strikingly unexpected transitional dynamics of Bose–Einstein magnon condensate: the density of the condensate increases immediately after the external magnon flow is switched off and initially decreases if it is switched on again. This behaviour finds explanation in a nonlinear ‘evaporative supercooling’ mechanism that couples the low-energy magnons overheated by pumping with all the other thermal magnons, removing the excess heat, and allowing Bose–Einstein condensate formation. Bose–Einstein condensation (BEC) [1] is achieved either by decreasing the temperature of an ideal gas of bosons [2] , or by increasing its density [3] , [4] . These two methods are valid for real atoms and molecules [5] , [6] as well as for gases of quasi-particles (QPs) such as, excitons [7] , polaritons [8] , [9] , [10] , magnons [11] , [12] , [13] and spatially confined photons [14] . In a gas in thermal equilibrium containing a fixed number of real atoms, the reduction of temperature leads to both the reduction of the average energy k B T of atoms and to the increase of the fraction of low-energy atoms in the energy distribution (see Fig. 1a ). In contrast, a QP gas most often does not have a fixed number of particles due to interaction with other subsystems, and thus cooling of an equilibrium QP gas results in the reduction of low-energy QP populations. A large concentration of low-energy QPs can be achieved artificially by external injection of QPs in a localized region of the spectrum where the QP energy is low (see Fig. 1b ). The resulting distributions in the energy of the particles and QPs ( Fig. 1a,b ) look remarkably similar, and the experiments show that BEC is possible in both above-described cases [5] , [6] , [11] , [14] . 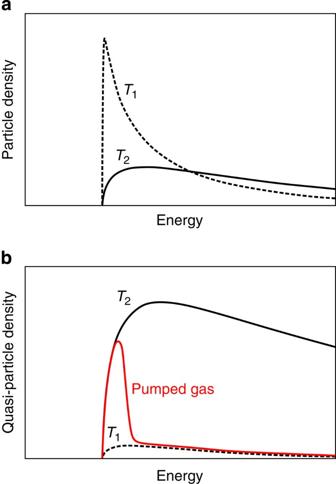Figure 1: Schematic energy distribution. (a) For an equilibrium system, containing a fixed number of real bosonic particles (atoms) and having chemical potential dependent on the temperature, at two different temperaturesT1<T2; (b) for an equilibrium system of bosonic QPs with zero chemical potential at two different temperaturesT1<T2(black curves). The red curve shows the non-equilibrium energy distribution of QPs in the case of external pumping in a low-energy part of the spectrum. It is clear, that the low-temperature distribution of atoms (black dashed curve corresponding toT1inFig. 1a) is qualitatively similar to the non-equilibrium distribution of QPs in the case of pumping in the low-energy part of the QP spectrum (red curve inFig. 1b). Figure 1: Schematic energy distribution. ( a ) For an equilibrium system, containing a fixed number of real bosonic particles (atoms) and having chemical potential dependent on the temperature, at two different temperatures T 1 < T 2 ; ( b ) for an equilibrium system of bosonic QPs with zero chemical potential at two different temperatures T 1 < T 2 (black curves). The red curve shows the non-equilibrium energy distribution of QPs in the case of external pumping in a low-energy part of the spectrum. It is clear, that the low-temperature distribution of atoms (black dashed curve corresponding to T 1 in Fig. 1a ) is qualitatively similar to the non-equilibrium distribution of QPs in the case of pumping in the low-energy part of the QP spectrum (red curve in Fig. 1b ). Full size image Of course, the first case corresponds to an equilibrium state of non-interacting bosons, while in the second case the QP distribution in energy is strongly non-equilibrium, and QPs are strongly interacting through scattering on each other. The strength and type of interactions between QPs can depend on the QP parameters, such as wavenumber (for magnons see, for example, refs 15 , 16 ), but this very interaction leads to a fast thermalization of the injected QPs (timescale of the order of 100 ns) [17] . Once a certain critical concentration of QP is reached, a BEC is established at the lowest energy state of the spectrum [17] , [18] , [19] . For magnons—the QPs of magnetic excitations (spin waves) of magnetically ordered media—injection of low-energy QPs is readily achieved via parametric microwave pumping [20] , [21] , making magnon systems valuable model environments for the study of general QP BEC dynamics. Until now, all the studies of QP BECs have implicitly assumed that the injected particles thermalize over the entire QP spectrum and that the sole role of the pumping is to increase the QP density, and thus the chemical potential of the QP gas. Here, we show that such a viewpoint is a crude oversimplification. Our observations of the transitional dynamics of gaseous and condensed (BEC) components of a pumped magnon gas are qualitatively incompatible with a uniform thermalization model. We show that, instead, the pumped magnons must thermalize and create a quasi-equilibrium state mainly in a narrow spectrally localized low-energy part of the magnon spectrum. This quasi-equilibrium spectral region can be characterized simultaneously by a very low average magnon energy (of the order of the energy of pumped magnons) and a very high effective temperature (defined as a temperature of the equilibrium gas of QPs having the same number of QPs in the narrow spectral region where the pumped quasi-equilibrium state is established (see Fig. 1b )), and that this quasi-equilibrium spectral region is coupled to the room-temperature magnon bath via a nonlinear supercooling mechanism. Dynamics of parametrically populated magnon gas Our experiments were performed on a magnon QP BEC system. Our sample comprised an in-plane magnetized Y 3 Fe 5 O 12 (YIG (yttrium-iron garnet)) film of 5 μm thickness grown on a Gd 3 Ga 5 O 12 (GGG) substrate (surface normal parallel to the <111> crystallographic axis). The scattering processes, which are responsible for magnon thermalization in YIG (a ferromagnetic insulator [22] , [23] ), take place on a timescale of 10–100 ns. This is significantly faster than the characteristic spin–lattice relaxation time, which is typically 400 ns. YIG’s uniquely long relaxation time makes it an exceptional model system for the investigation of general QP BECs. In our experiments, high magnon densities were created using the well-established technique of parallel parametric pumping [20] , [21] . The pumping process involves the splitting of microwave photons from the pumping field (oriented parallel to the static magnetization of the sample) into pairs of magnons having one-half of the pump frequency and oppositely oriented wavevectors. 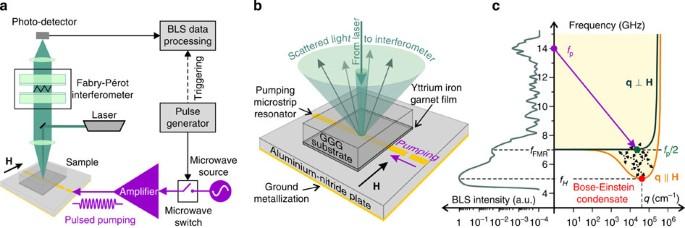Figure 2: Set-up for excitation and observation of magnons. (a,b) The YIG film sample is placed above a microstrip pump resonator prepared on top of a metallized AlN plate. A bias magnetic fieldHof 1,735 Oe is applied in the film plane across the resonator. The resonator is driven by microwave pulses of carrier frequencyfp=14 GHz. A probing laser beam is focused onto the microstrip. The scattered light is directed to a Fabry–Pérot interferometer for analysis. (c) The measured frequency spectrum of the inelastically scattered light (left) is presented in relation to the magnon spectrum (right, yellow shaded area). The curves on the right abscissa show the dispersion relations for magnons with wavevectorsqlying in the film plane across (dark green) and along (orange) the bias magnetic fieldH. The yellow shaded area contains the dispersion relations for magnons propagating in every direction in the film. The purple arrow illustrates the creation of primary magnons (green dot) by parametric pumping (purple dot). The dashed arrows schematically represent the thermalization of the parametrically injected magnons. The highest intensity BLS peak is associated with the BEC at the lowest energy state (red dot) at frequencyfH=5 GHz and wavenumberq=4 × 104cm−1. The second BLS intensity maximum at frequencyfp/2 is created by the parametrically injected magnons, while the third at frequencyfpresults from non-resonant magnetization precession directly forced by the pumping field.fFMRis the ferromagnetic resonance frequency. Figure 2a shows a sketch of our experimental set-up. A continuous wave generated by a microwave source at a frequency of f p =14 GHz is chopped by a fast microwave switch into a sequence of rectangular shaped pump pulses of 2 μs duration having sharp edges of 3 ns width. The switch itself is driven by a pulse generator. After amplification up to 25 W, the pulses are sent to the YIG film (see Fig. 2b ). The pumping field is applied to the YIG film via a 50 μm-wide microstrip resonator directly processed onto the surface of a high thermal conductivity aluminium-nitride dielectric plate. On account of this design, a repetition time of 100 μs is sufficiently low to reduce the average pumping power to a level at which the influence of microwave heating on the experimental data can be excluded. The temporal dynamics of the magnon gas was investigated with a resolution of about 1 ns by means of time-resolved Brillouin light scattering (BLS) spectroscopy [24] . The YIG sample was probed by a coherent optical beam of wavelength 532 nm and power ~0.5 mW. The low light intensity was specifically chosen to avoid unwanted heating of the probing point. Figure 2: Set-up for excitation and observation of magnons. ( a , b ) The YIG film sample is placed above a microstrip pump resonator prepared on top of a metallized AlN plate. A bias magnetic field H of 1,735 Oe is applied in the film plane across the resonator. The resonator is driven by microwave pulses of carrier frequency f p =14 GHz. A probing laser beam is focused onto the microstrip. The scattered light is directed to a Fabry–Pérot interferometer for analysis. ( c ) The measured frequency spectrum of the inelastically scattered light (left) is presented in relation to the magnon spectrum (right, yellow shaded area). The curves on the right abscissa show the dispersion relations for magnons with wavevectors q lying in the film plane across (dark green) and along (orange) the bias magnetic field H . The yellow shaded area contains the dispersion relations for magnons propagating in every direction in the film. The purple arrow illustrates the creation of primary magnons (green dot) by parametric pumping (purple dot). The dashed arrows schematically represent the thermalization of the parametrically injected magnons. The highest intensity BLS peak is associated with the BEC at the lowest energy state (red dot) at frequency f H =5 GHz and wavenumber q =4 × 10 4 cm −1 . The second BLS intensity maximum at frequency f p /2 is created by the parametrically injected magnons, while the third at frequency f p results from non-resonant magnetization precession directly forced by the pumping field. f FMR is the ferromagnetic resonance frequency. Full size image The measurement arrangement is illustrated in Fig. 2b . The focused incident laser beam passes through the film, scatters from the pumping resonator and, on the way back, inelastically scatters from magnons in the YIG before being collected and sent to a multi-pass tandem Fabry–Pérot interferometer. The frequency shift and intensity of the scattered light are a measure of the magnon frequency and density, respectively. The frequency spectrum of the scattered light measured in our experiments is shown in Fig. 2c in relation to the simplified spectrum of magnons in the YIG. The BLS peak observed at 7 GHz is caused by magnons excited directly through the microwave field of the pumping resonator at one-half of the pumping frequency. By adjusting the magnetizing field H to 1,735 Oe, this frequency is close to the ferromagnetic resonance frequency f FMR . The magnons parametrically injected at 7 GHz thermalize via multistage four-magnon scattering processes to the bottom of the magnon spectrum f H where they give rise to a BLS peak near 5 GHz. 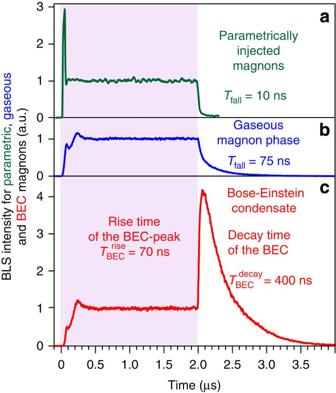Figure 3: Time evolution of the magnon density. The BLS intensity is proportional to the magnon density. BLS measurements were performed in frequency windows of 150 MHz around 7, 6 and 5 GHz. The purple area indicates the time over which the pump is active. (a) Parametrically injected magnons at 7 GHz. The sharp peak at the front of the pulse is due to transient processes in the system of parametrically excited magnons21,25. (b) Gaseous magnon phase lying between the region of parametrically injected magnons and the bottom of the magnon spectrum (6 GHz). (c) BEC at the bottom of the magnon spectrum (5 GHz). The decay of the parametrically injected (primary) and gaseous magnons after the end of the pumping pulse is non-exponential. The indicated fall times correspond to 50% decay. Note that the rise time of the dramatic jump in the density of the condensed magnons is well correlated with the decay of the gaseous magnons. Figure 3a shows the time evolution of the BLS intensity for magnons at one-half of the pumping frequency. The purple shaded area indicates the time over which the pumping is enabled. The sharp peak at the beginning of the pumping is due to transient processes and is an artefact of the parametric pumping mechanism [21] , [25] . Figure 3: Time evolution of the magnon density. The BLS intensity is proportional to the magnon density. BLS measurements were performed in frequency windows of 150 MHz around 7, 6 and 5 GHz. The purple area indicates the time over which the pump is active. ( a ) Parametrically injected magnons at 7 GHz. The sharp peak at the front of the pulse is due to transient processes in the system of parametrically excited magnons [21] , [25] . ( b ) Gaseous magnon phase lying between the region of parametrically injected magnons and the bottom of the magnon spectrum (6 GHz). ( c ) BEC at the bottom of the magnon spectrum (5 GHz). The decay of the parametrically injected (primary) and gaseous magnons after the end of the pumping pulse is non-exponential. The indicated fall times correspond to 50% decay. Note that the rise time of the dramatic jump in the density of the condensed magnons is well correlated with the decay of the gaseous magnons. Full size image After the pumping is switched off, the intensity of the directly injected magnons rapidly decays as a result of strong four-magnon scattering. The fall time of this peak (10 ns) can be used as a rough estimate of the thermalization time of the magnon gas. The gaseous magnon phase, which lies between the region of the parametrically injected magnons and the bottom of the magnon spectrum, also decays after the pumping pulse ends (see Fig. 3b ). This decay is very clearly non-exponential and happens on a much longer timescale (75 ns) than the thermalization of the primary injected magnons. Interestingly, the BEC at the bottom of the spectrum is found to exhibit a different, unexpected behaviour when the pumping is switched off. As shown in Fig. 3a,c a dramatic upward jump in the density of the condensed magnons is observed, which is correlated in its timing with the fall in density of the gaseous magnon phase. After reaching a peak density, the condensate then decays with the spin–lattice relaxation time of about 400 ns. Spectrally localized heating The surprising dynamics we observe can be understood qualitatively by considering a simple picture of the thermalization of a parametrically driven QP gas. The parametric pumping process creates a constant flow of magnons at the injection frequency f in = f p /2 (see Fig. 4a ). For the spectral region under consideration (and for the chosen magnitude of the magnetizing field), the direct scattering of the injected magnons to the lowest energy states, which would conceal the BEC phenomenon, is prohibited by energy and momentum conservation laws [20] . Thus, the injected magnons scatter via four-magnon processes—multistage events that are localized in energy space—and a quasi-equilibrium state of the pumped magnon gas is reached. Due to the fact that these magnon scattering processes are localized in a particular energy region [26] , the quasi-equilibrium condition is established only over a finite region of the magnon spectrum: all states from the bottom of the spectrum ε min = hf H (where h is the Planck constant) to a certain maximum energy ε max = hf max are in a thermal quasi-equilibrium characterized by an effective temperature T and chemical potential μ . The rest of magnons ( ε > ε max ) are unaffected and reside at room temperature and at zero chemical potential. Since all relevant energies of the pumped magnons are much smaller than the room-temperature thermal energy (for example, the characteristic temperature for the injection frequency f in =7 GHz is ε in / k B = hf in / k B =0.34 K), we assume ε max << k B T . 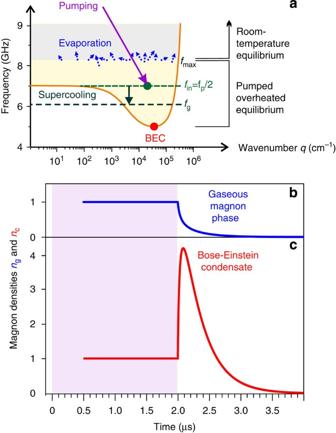Figure 4: Supercooling of the magnon gas and transitional dynamics of the BEC. (a) A schematic illustration of the evaporative supercooling process. The purple arrow shows the incoming flow of parametrically injected magnons with frequencyfin=fp/2 to the region of the magnon gas spectrum (shaded in yellow) corresponding to the pumped overheated equilibrium. The small dashed arrows indicate nonlinear scattering (‘evaporation’) of high-energy magnons having frequencies near the upper edge of the ‘pumped’ regionfmaxto undisturbed states in the ‘room-temperature’ region of the magnon spectrum. The downward black arrow represents the decrease of the average energyhfgof the pumped gaseous phase (‘supercooling’) as a result of this evaporation.his Planck’s constant. The red dot marks the position of the BEC. (b,c) Calculated transitional dynamics of the gaseous magnons from the pumped area and the condensed magnons.ngis the density of the gaseous magnon phase in the ‘pumped’ region,ncthe density of the BEC. The purple shaded area indicates the time over which the pump is active.ngandncare normalized to their steady-state values during pumping. In this high-temperature limit, the population (number) density n ( ε ) of the pumped magnons is described by the Rayleigh–Jeans distribution: Figure 4: Supercooling of the magnon gas and transitional dynamics of the BEC. ( a ) A schematic illustration of the evaporative supercooling process. The purple arrow shows the incoming flow of parametrically injected magnons with frequency f in = f p /2 to the region of the magnon gas spectrum (shaded in yellow) corresponding to the pumped overheated equilibrium. The small dashed arrows indicate nonlinear scattering (‘evaporation’) of high-energy magnons having frequencies near the upper edge of the ‘pumped’ region f max to undisturbed states in the ‘room-temperature’ region of the magnon spectrum. The downward black arrow represents the decrease of the average energy hf g of the pumped gaseous phase (‘supercooling’) as a result of this evaporation. h is Planck’s constant. The red dot marks the position of the BEC. ( b , c ) Calculated transitional dynamics of the gaseous magnons from the pumped area and the condensed magnons. n g is the density of the gaseous magnon phase in the ‘pumped’ region, n c the density of the BEC. The purple shaded area indicates the time over which the pump is active. n g and n c are normalized to their steady-state values during pumping. Full size image Time traces of magnon populations at intermediate energies ε in > ε > ε min ( Fig. 3b ) allow us to estimate the effective temperature T . Using equation (1), the increase in the driven magnon population when the BEC is formed ( μ = ε min ) relative to its room-temperature density ( T =300 K, μ =0) can be written as follows: where ε /( ε — ε min ) describes the increase in the density of the gaseous magnon phase due to an increase in the chemical potential μ alone. For the data of Fig. 3b ( ε / h =6 GHz, ε min / h =5 GHz) ε /( ε — ε min )~6 and equation (2) gives In our experiments, the room-temperature population n 0 ( ε ) was close to the background noise level ( n 0 ( ε )=0.0015 on the scale used in Fig. 3b ). Accordingly, the density of the gaseous magnon phase is seen to increase 666 times during the pumping pulse, implying that the effective temperature of the pumped magnon gas is T ≈30,000 K. This estimate might at first seem unreasonably high, however, it is important to realize that the high effective temperature exists only in a very small region ( ε max > ε > ε min ) of the magnon gas’ phase space, and, as such, has very little influence on its aggregate parameters (such as, for example, the total number of magnons). Thus, the magnon BEC evolves in a very narrow spectral region, which is strongly overheated by the pumping. Evaporative supercooling Besides the parametric injection and thermalization processes, the dynamics of the overheated pumped region are influenced by spin–lattice relaxation (which reduces the number of magnons with an energy-independent frequency Γ), and the scattering of magnons into higher energy states (which provides coupling between the overheated quasi-equilibrium low-energy magnons and the rest of the magnon spectrum). The latter process is analogous to the evaporative cooling process of a real gas [27] : magnons with highest energies leave the quasi-equilibrium region, thus reducing the average magnon energy from the injection energy hf in to a lower value hf g < hf in (see Fig. 4a ). In the case of high-temperature QP gases in which the thermal energy k B T is larger than the characteristic energy hf max of the local equilibrium, the evaporation is especially efficient and leads not only to a reduction of the effective temperature T , but also to an increase of the chemical potential μ (see Methods): the process can be considered as nonlinear evaporative supercooling. Evaporative supercooling of the magnon gas provides a convincing qualitative explanation of the formation of the pronounced BEC peak after the pumping is switched off ( Fig. 3c ). During the action of the pumping, energy losses due to evaporative supercooling are balanced by ‘heating’ of the magnon gas by the injected magnons (since hf in > hf g ). When the pumping ceases, evaporation of magnons continues, leading to a net reduction in the average magnon energy and thus to an increase in the condensed fraction of the magnon gas. A comparison of the physical picture outlined above with the experimental findings can be performed using a simple model describing the dynamics of the quasi-equilibrium in the overheated QP gas where the BEC phase has been already formed (see Methods for further details). This model can be applied to any pumped QP system with a local equilibrium. When the chemical potential in the QP gas reaches the minimum QP energy hf min , the BEC phase is established and the thermodynamic state of the quasi-equilibrium region ( ε max > ε > ε min ) can be described in terms of a normalized number of particles in the condensed ( n c ) and gaseous ( n g ) phases. The equations describing the dynamics of n c and n g can be derived by considering rate equations for the total number and total energy of particles in the quasi-equilibrium region: Here, the QP relaxation rate Γ sets the overall characteristic timescale of the transitional dynamics (in the case of magnons, Γ describes magnon–phonon relaxation). The first terms on the right-hand sides of equation (4) describe injection of QPs by time-dependent pumping n in ( t ). The coefficient λ (defined in Methods by equation (16)) lies between 0 and +1, and depends on the injection energy hf in and the parameters of the quasi-equilibrium region in the QP gas. The middle terms on the right-hand sides of equation (4) describe linear QP relaxation, and the final one, the nonlinear evaporative supercooling of the QP gas via four-particle scattering involving higher energy states ( ε > ε max ). Note that the nonlinear scattering of particles within the region ε max > ε > ε min does not enter equation (4) explicitly because such processes change neither the total number nor the total energy of the QPs in the thermalized region. We stress that, so long as conditions of local quasi-equilibrium are satisfied, equation (4) can be applied to any system of QPs with linear relaxation, external particle injection and four-particle scattering. The specific features of a particular system (for instance, density of QP states) determine only the normalization of the particle densities n c and n g and the dimensionless coefficient λ . In other words, though quantitative aspects of the transient dynamics of a particular QP BEC depend on the value of λ , the qualitative picture remains the same. It should be noted that for λ >0, the direct contribution of the injection flux n in ( t ) into the equation for the BEC density n c is negative. This is due to the fact that, as alluded to above, the pumping injects QPs with energies higher than the average QP energy and therefore heats the gas. In contrast, the evaporation contribution ( ) in the BEC equation has a positive sign since it reduces the average QP energy and therefore increases the BEC density. The results of calculations based on the model of equation (4) for the conditions corresponding to our experiments ( Fig. 3 ) are shown in Fig. 4b,c . After the end of the pumping pulse, a large peak in the BEC density with an amplitude and duration very similar to that observed in our experiments is clearly seen. At the same time, the gaseous fraction of the magnon gas n g decays monotonically. Since both are caused by the same evaporative process, the growth time of the BEC peak is well correlated with the decay time of the gaseous magnons. BEC density reduction by magnon injection The model of equation (4) predicts a further surprising dynamic property of the overheated QP BEC: an initial rapid decrease in the density of a freely decaying BEC ( n in =0) in response to pumping (see model calculations in Fig. 5a,b ). The reason for this pumping-induced destruction of the BEC is that the pumping injects QPs having energy hf in , which is above the average QP energy hf g . In the absence of the evaporative supercooling (which requires some time to fully develop), the only means by which this excess energy can be absorbed is for particles from the BEC to move into the gaseous phase, reducing the condensate density. This prediction has been verified experimentally using a sequence of two pumping pulses (see experimental curves in Fig. 5a,b ). A first long pumping pulse was used to establish an overheated magnon BEC. After the end of this pulse, the density of the gaseous magnons was observed to decrease through relaxation and evaporation, while an initial BEC peak—similar to the one recorded in Fig. 3c and Fig. 4c—was formed. A second pumping pulse was applied 100 ns after the end of the first one. Immediately after the start of this second pump, the BEC density was observed to rapidly decrease at a rate perfectly correlated with a corresponding increase in the gaseous fraction. The growth of the BEC density towards its equilibrium value (reached at 300 ns) begins only after the gaseous fraction has increased and evaporative supercooling has established. The simple model of equation (4) (solid line in Fig. 5 ) describes all the qualitative features of the experiment remarkably well. 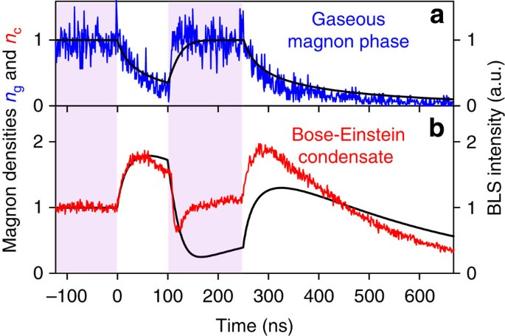Figure 5:Pump-induced destruction of aQPBEC. The purple shaded areas indicate the action times of two pump pulses. The first creates an overheated magnon gas where the pumped equilibrium is established and the BEC is formed. The second is used to probe the free evolution of the magnon gas. (a) Theoretical prediction of evolution of the density of the gaseous magnon phasengin the pumped equilibrium region (black solid curve) and corresponding BLS data measured at 6 GHz between the region of parametrically injected magnons and the bottom of the magnon spectrum. (b) Theoretical prediction of evolution of the density of the condensed magnon phasenc(black solid curve) and BLS data corresponding to the magnon BEC. Note the immediate and simultaneous increase of the magnon gas density and decrease of the BEC density after the second pump pulse is switched on. The faster than predicted growth of densities of both the gaseous phase and BEC during the action of the second pump pulse is caused by the transitional processes in pumping (see the sharp peak at the beginning of the pumping pulse inFig. 3aand the corresponding humps inFig. 3b,c, as well as the additional description in Methods). For the same reason, the intensity of the experimentally observed second BEC peak exceeds the intensity of the first one. Figure 5: Pump-induced destruction of a QP BEC. The purple shaded areas indicate the action times of two pump pulses. The first creates an overheated magnon gas where the pumped equilibrium is established and the BEC is formed. The second is used to probe the free evolution of the magnon gas. ( a ) Theoretical prediction of evolution of the density of the gaseous magnon phase n g in the pumped equilibrium region (black solid curve) and corresponding BLS data measured at 6 GHz between the region of parametrically injected magnons and the bottom of the magnon spectrum. ( b ) Theoretical prediction of evolution of the density of the condensed magnon phase n c (black solid curve) and BLS data corresponding to the magnon BEC. Note the immediate and simultaneous increase of the magnon gas density and decrease of the BEC density after the second pump pulse is switched on. The faster than predicted growth of densities of both the gaseous phase and BEC during the action of the second pump pulse is caused by the transitional processes in pumping (see the sharp peak at the beginning of the pumping pulse in Fig. 3a and the corresponding humps in Fig. 3b,c , as well as the additional description in Methods). For the same reason, the intensity of the experimentally observed second BEC peak exceeds the intensity of the first one. Full size image We have presented and experimentally verified a new physical picture of local thermalization in a gas of QPs strongly overpopulated by external pumping. In this case, the spectral non-uniformity of the QPs distribution function can be interpreted as a spectrally non-uniform temperature [28] , [29] . In the experimental case of a parametrically pumped magnon gas, the thermalization of QPs occurs only over a very narrow spectral interval encompassing the lowest energy states, and the formation of a magnon BEC takes place in a strongly overheated spectral area having an effective temperature exceeding 30,000 K. The work also reveals the key physical mechanism which underpins the formation of a QP BEC at such high local effective temperatures. This is a mechanism that may be described as evaporative supercooling of QPs which brings about the reduction in their average energy, increases the chemical potential of the QP gas and provides coupling with the rest of the thermal magnons. The evaporative supercooling mechanism has a profound influence on the transitional dynamics to the condensate: notably, the BEC density increases when the pumping is switched off and vice versa. The validity of the evaporative cooling theory of a hot BEC is convincingly corroborated by our measurements of the time evolution of a BEC of magnons in wavenumber space ( Fig. 6 ). Since the dispersion curve of the low-energy magnons is very flat (the wavenumber q varies here from 10 4 to 10 5 cm −1 in a frequency band of 150 MHz, which usually corresponds to the resolution of the Fabry–Pérot interferometer, see Fig. 3a ), wavenumber distribution measurements are necessary to confirm the existence of the condensed magnon state [30] . These measurements were performed using a rotating sample stage as described in ref. 31 with a wavenumber resolution Δ q ≅ 0.4 × 10 4 cm −1 . In the case of a low pumping power of 1 W—corresponding to the case of a moderate heating of the magnon gas—a clear concentration of magnons occurs at the global energy minimum (compare Figs 4a and 6a ) q =4 × 10 4 cm −1 . For a high pumping power of 25 W, the magnon gas is too hot for BEC to occur during the pumping pulse and the condensate only appears as a result of evaporative supercooling after the pump has been switched off ( Fig. 6b ). We stress that the post-pumping increase in condensed magnon density we observe cannot be caused by conventional cooling of the magnon gas of the kind observed, for example, in exciton gases uniformly overheated by injection of hot ( hf in > k B T ) QPs [7] . In contrast to ref. 7 , we pump very cold magnons with energies corresponding to temperatures much lower than the ambient temperature. 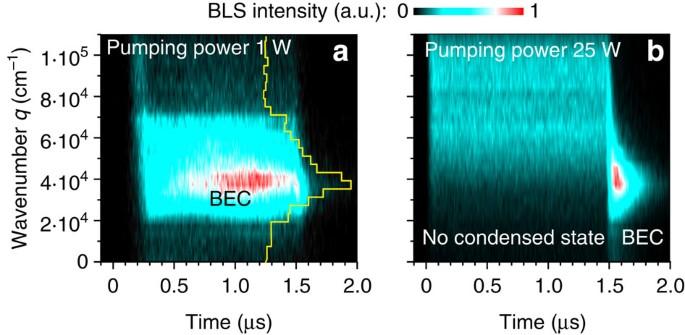Figure 6: Time evolution of the BEC of magnons in wavenumber space. The pump pulse of 1.5 μs duration is switched on at zero time. The BLS intensities are measured in a frequency band of 150 MHz near the bottom of the magnon spectrum for different magnon wavevectorsqalong the magnetization direction. (a) In the case of a relatively low pumping power, the parametrically injected magnons thermalize in energy–wavevector space, populate the bottom of the magnon spectrum and create a BEC at the global energy minimum near the wavenumberq=4 × 104cm−1. The yellow histogram shows the dependence of the BLS intensity on the wavenumberq1.24 μs after the pumping starts. The narrow BEC peak is clearly visible on the background of the broad gaseous hump. (b) In the case of a strong pumping and, consequently, of a significantly overheated magnon gas the magnon BEC does not form during the pumping pulse, but appears as a result of the evaporative supercooling after the pump is switched off. Figure 6: Time evolution of the BEC of magnons in wavenumber space. The pump pulse of 1.5 μs duration is switched on at zero time. The BLS intensities are measured in a frequency band of 150 MHz near the bottom of the magnon spectrum for different magnon wavevectors q along the magnetization direction. ( a ) In the case of a relatively low pumping power, the parametrically injected magnons thermalize in energy–wavevector space, populate the bottom of the magnon spectrum and create a BEC at the global energy minimum near the wavenumber q= 4 × 10 4 cm −1 . The yellow histogram shows the dependence of the BLS intensity on the wavenumber q 1.24 μs after the pumping starts. The narrow BEC peak is clearly visible on the background of the broad gaseous hump. ( b ) In the case of a strong pumping and, consequently, of a significantly overheated magnon gas the magnon BEC does not form during the pumping pulse, but appears as a result of the evaporative supercooling after the pump is switched off. Full size image The experiments presented in this article were performed using a parametrically pumped QP gas of magnons. However, our key findings may be generalized to any low-energy ( hf << k B T ) system of interacting QPs, and the unusual transitional BEC dynamics we observe should, in principle, be observable in pumped systems of excitons, polaritons and photons. In conclusion, our results demonstrate that the temperature of the thermal bath (in our case 300 K) is not an important factor in the formation of a QP BEC, since the local temperature of the quasi-equilibrium gas of QPs overheated by pumping is much larger ( T ≈30,000 K in our experiments). It is this overheated gas of QPs that dominates the dynamics of the system, leading to the formation of BEC. The new physical interpretation of QP BEC formation we present here also suggests new ways to control the formation of QP BECs by enhancing or suppressing the process of evaporative supercooling. This might be achieved, for example, through the use of metamaterials [32] having specially designed densities of states. Samples The magnon gas dynamics reported here were reproducibly observed in a variety of samples of in-plane magnetized YIG (Y 3 Fe 5 O 12 ) films of different thickness (2–7 μm) and lateral sizes (a few square millimetres) grown in the (111) crystallographic plane by liquid phase epitaxy on gallium gadolinium garnet substrates Gd 3 Ga 5 O 12 and having a saturation magnetization of around 1,750 G. The magnon spectrum in such samples is strongly anisotropic relative to the angle between the magnetic bias field H and magnon wavevector q [33] . In the case of longitudinally propagating magnons ( q || H ), the competitive contributions of exchange and dipolar inter-spin interactions result in a non-monotonic relation between magnon energy and momentum (see Fig. 2c ) that results in a global energy minimum at f H = γH , where γ =2.8 MHz/Oe is the electron gyromagnetic ratio. For a magnetizing field of H =1,735 Oe (as employed in our experiments), this minimum ( f H =5 GHz) lies significantly above the half frequency of the injected magnons ( f in /2=3.5 GHz), and thus three-magnon splitting is prohibited by energy conservation. As a result, only two- and four-particle scattering processes, which conserve the total magnon number, contribute to thermalization. Parametric parallel pumping Parametric pumping is the most effective method of magnon injection. In contrast with forced resonant excitation of magnetization precession—which is widely used in ferromagnetic resonance measurements—the density of parametrically excited magnons cannot be restricted by linear damping. This is because parametric energy transfer is proportional not only to the amplitude of the pumping field but also to the QP density. As soon as the magnetic losses are compensated by the applied pumping, the magnon density increases exponentially in time until it is limited by nonlinear mechanisms [20] . As the limiting processes involved need a finite time to fully develop [34] , a high peak of injected magnon density can be clearly observed after the front of the pumping pulse (see Fig. 3a ). In our experiment, we use first-order parametric excitation in which one photon of the microwave magnetic field, which is induced around a microstrip resonator parallel to the bias field H , splits into two magnons at half of the pumping frequency f p . To begin with, all magnon states at f p /2 are populated but, due to the competition between magnon modes, only the magnon group most strongly coupled with the pumping field survives to the steady-state regime [20] . Above the ferromagnetic resonance frequency, this group belongs to the transverse magnon branch ( q ⊥ H ) [35] . Transverse magnons, which propagate along the pumping microstrip, do not leave the pumping area and thus absorb the pumping energy most effectively [36] . A narrow (50 μm width) half-wavelength (~3 mm length) microstrip resonator with loaded quality factor Q =25 at f p =14 GHz is used to increase the pumping field amplitude through accumulation of the pumping energy and spatial concentration of the pumping field. At the same time, the moderate quality factor of a pumping resonator enables fast (nanosecond timescale) ‘on’ and ‘off’ switching of pumping. Wavevector resolved BLS spectroscopy The maximum efficiency of inelastic light scattering is reached for magnons which satisfy the Bragg condition q =2 q light sin( θ ), where θ is the angle between the wavevector of the probing light q light and the magnon wavevector q lying in the sample plane. Thus, the wavevector selectivity of magnons can be achieved by rotating the sample relative to the probing laser beam. To ensure constant magnetization conditions in the case of q || H , the sample together with the whole magnet assembly are rotated simultaneously. Due to geometrical constraints of the rotating stage, the magnons are detected up to q =1.1 × 10 5 cm −1 with wavenumber resolution of Δ q ≃ 0.4 × 10 4 cm −1 (ref. 31 ). The frequency resolution of our BLS measurements is 150 MHz. Local thermalization in a pumped magnon gas We postulate that the magnon states from the lowest magnon energy ε min = hf H to a certain maximum energy ε max = hf max reside in a pumped thermodynamic equilibrium with effective temperature T and chemical potential μ , while the rest of magnons ( ε > ε max ) are unaffected. The high temperature (T~30,000 K in our experiments) and high relative density of pumped magnons allows scattering of room-temperature magnons into the pumped region to be completely neglected. However, the inverse process—scattering of pumped magnons into higher energy states—becomes extremely significant since its intensity increases with that of the magnon density n ( ε ); this scattering process is of crucial importance for the formation of the BEC. We note that the effects of stimulated magnon scattering are implicitly taken into account in our consideration since we assume that the equilibrium distribution of magnons in the relevant low-energy spectral region is of the quantum Bose–Einstein type and the processes of stimulated magnon scattering determine the difference between the quantum Bose–Einstein distribution and the classical Maxwell–Boltzmann distribution. A model of the transitional dynamics of a pumped magnon gas can be developed based on the rate equations for the total number N and total energy E of the magnons in the pumped region ε max > ε > ε min . For simplicity, we restrict our discussions to the situation in which the magnon BEC has already formed. In this case, the chemical potential μ is fixed at μ = ε min and the thermodynamic state of the pumped magnons is characterized by an effective temperature T and the number of condensed (BEC) magnons N c . The total number of magnons N is where N g is the number of gaseous magnons in energy states ε max > ε > ε min . Using equation (1), N g can be written as follows: where D ( ε ) is the density of magnon states. The energy of the pumped magnons can also be split into condensed and gaseous parts: Since each condensed magnon has the same energy ε min , the BEC energy E c has a simple form: The energy of the gaseous fraction, E g , can be written as follows: where the average energy of gaseous magnons ε g is defined as Note, that so long as the cutoff energy ε max is temperature independent, the mean energy ε g is constant. Clearly, ε max > ε g > ε min . Note also that in the case when a BEC is not formed ( μ < ε min ), the average magnon energy (determined by equation (10) with substitution ε min → μ in the integrands) depends only on the chemical potential μ . This is in contrast with real gases, where the mean energy depends chiefly on the temperature T . This difference is due to the fact that while magnons are low-energy excitations, for which ( ε — μ ) << k B T and equation (10) is valid approximately, real gases generally inhabit the opposite limit ( ε — μ ) >> k B T , where the Bose–Einstein distribution can be approximated by the Boltzmann distribution. The rate equations for the number of magnons N and magnon energy E can be written as follows: The first term in the right-hand side of equation (11) describes injection of magnons by parametric pumping. J in ( t )≥0 is the time-dependent rate of injection and ε in is the energy of the injected magnons. The second term describes spin–lattice relaxation of the overheated magnons. Due to the high temperature (or large magnon density) in the pumped region, magnon excitation by lattice vibrations (incoming terms of the form +Γ N 0 ) are neglected. The spin–lattice relaxation rate is assumed constant in the energy range ε max > ε ≥ ε min , resulting in identical relaxations rate Γ for magnon number and energy. Note, that in terms of the thermodynamic parameters T and μ (see equation (1)), such relaxation is equivalent to the cooling of the magnon system, that is, it reduces the temperature T while the chemical potential μ remains unchanged. The last term in the right-hand side of equation (11) describes nonlinear scattering of the pumped magnons into higher energy states (that is, into the region of room-temperature equilibrium). Since the scattering processes are approximately localized in energy space, the intensity of this scattering (two pumped magnons scatter into one magnon in the pumped regime ε max > ε > ε min and one magnon in the room-temperature regime ε > ε max ) is proportional to [ n ( ε max )] 3 , that is, to N g 3 . Each magnon that leaves the overheated region takes with it an energy ε ≈ ε max , hence the magnon number and energy fluxes differ by a factor ε max . The coefficient β is proportional to the four-magnon scattering coefficient. Note that the most intense scattering processes (scattering of two magnons in the pumped regime into two different states within the pumped regime) do not change either the number N or the energy E and therefore do not contribute to the rate (equation (11)). These processes lead to the thermalization of the overheated region and are implicitly taken into account by the thermal distribution (equation (1)). The scattering processes ( β ) find a parallel with the evaporative cooling of a real gas [15] : in both cases the highest energy particles leave the gas. However, in the magnon gas context such an evaporation process not only reduces the gas temperature (by reducing the number of QPs) but, also increases the chemical potential (by reducing their average energy). For this reason, the scattering might be regarded as a mechanism of supercooling. Since the spin–lattice relaxation does not change the average energy of magnons and evaporative supercooling reduces it, the mean energy ε g must be smaller than the injection energy ε in : This simple relation is of central importance for the transient dynamics of the magnon BEC. Equation (11) can be solved for the number of magnons in the condensed N c and gaseous N g fractions: This system can be written in a simpler form by introducing dimensionless magnon densities: a dimensionless injection rate: and dimensionless parameter: which lies between 0 and 1 and describes, in essence, the intensity of the supercooling process. In dimensionless form, the balance equations for n c and n g are shown by equation (4): We see that—perhaps rather unexpectedly—the pumping term acts to reduce the BEC density n c . The physical reason for this is clear from the previous analysis: the pumping injects magnons having energy ε in larger than the average magnon energy ε g (see equation (12)). Without evaporative supercooling, the only way to absorb this excess energy is to move part of the BEC magnons into the gaseous phase, thus reducing the BEC density. In contrast, evaporative supercooling—which reduces the average magnon energy—acts to increase n c . Equation (4) provide an explanation for the appearance of the BEC peak after the pumping is switched off (see Fig. 3c ). When the pumping is acting, a stationary state is established with Immediately after the pumping is switched off, the magnon densities n c and n g stay the same and we have The model of equation (4) also predicts that a free-decaying BEC will initially reduce its intensity dn c / dt <0 in response to pumping before a new driven stationary regime is established. The theoretical curves shown in Figs 4 and 5 were calculated by solving equation (4) numerically with the following parameters: Γ=3.1 μs –1 , n in =2.34, λ =0.83 for Fig. 4 and Γ=3.1 μs –1 , n in =2.67, λ =0.83 for Fig. 5 . How to cite this article: Serga, A. A. et al. Bose–Einstein condensation in an ultra-hot gas of pumped magnons. Nat. Commun. 5:3452 doi: 10.1038/ncomms4452 (2014).